Direct imaging of single UvrD helicase dynamics on long single-stranded DNA Fluorescence imaging of single-protein dynamics on DNA has been largely limited to double-stranded DNA or short single-stranded DNA. We have developed a hybrid approach for observing single proteins moving on laterally stretched kilobase-sized ssDNA. Here we probed the single-stranded DNA translocase activity of Escherichia coli UvrD by single fluorophore tracking, while monitoring DNA unwinding activity with optical tweezers to capture the entire sequence of protein binding, single-stranded DNA translocation and multiple pathways of unwinding initiation. The results directly demonstrate that the UvrD monomer is a highly processive single-stranded DNA translocase that is stopped by a double-stranded DNA, whereas two monomers are required to unwind DNA to a detectable degree. The single-stranded DNA translocation rate does not depend on the force applied and displays a remarkable homogeneity, whereas the unwinding rate shows significant heterogeneity. These findings demonstrate that UvrD assembly state regulates its DNA helicase activity with functional implications for its stepping mechanism, and also reveal a previously unappreciated complexity in the active species during unwinding. Single-stranded DNA (ssDNA) is an intermediate in various DNA metabolic processes, such as replication, repair and recombination, wherein a multitude of proteins bind to ssDNA and perform their functions in coordination with each other. The ssDNA binding proteins, recombinase proteins (RecA/Rad51) and DNA helicases/translocases are among the proteins that have an important function in genome maintenance, and the dynamics of these proteins on ssDNA have been studied at the single-protein level [1] . Although these assays have revealed a wealth of information on the details of ssDNA–protein interactions at the scale of tens of nucleotides [2] , [3] , [4] , [5] , [6] , there remains an interest in the dynamics on longer length scales, as ssDNA in the cell can be thousands of nucleotides long [7] , [8] . Thus, to better emulate the physiological situation it would be advantageous to study protein–DNA interactions at the single-protein level using long ssDNA molecules. Direct fluorescence imaging of proteins moving on long double-stranded DNA (dsDNA) has been demonstrated by many laboratories [9] , [10] , [11] , [12] , [13] . Yet, there has been no equivalent demonstration for protein dynamics on long ssDNA, although fluorescence imaging of proteins bound on ssDNA was recently reported [14] , [15] , [16] . One of the technical difficulties, which might have impeded imaging of proteins on ssDNA, is the high propensity for forming intra- and intermolecular base pairing in ssDNA. In a long ssDNA, numerous secondary structures can be formed by internal base pairing [17] unless the DNA is chemically denatured [18] . Such secondary structures can influence interpretations of experimental data obtained from the measurement of DNA end-to-end distances upon which most single-molecule force spectroscopy is based. Some of these secondary structures are transient, displaying opening and closing dynamics [19] , which adds unwanted noise to the measurement. On the other hand, hairpins with long duplex stems are very stable and almost always are in the closed state unless an unzipping force is applied [20] . Either these structures should be completely unzipped by applying high-enough forces or the formation of such structures should at least be monitored. Therefore, the capacity of mechanical manipulation is indispensable for analysing single-protein dynamics on long ssDNA. Here we combine total internal reflection fluorescence (TIRF) microscopy with optical tweezers and unzip all secondary structures within the ssDNA molecules by stretching. The exponentially decaying excitation profile of the TIRF microscopy selectively illuminates only the molecules within a few hundred nanometres from the surface and this enables the detection of single fluorophores with a high signal-to-noise ratio. An optical trap applies force to DNA substrates tethered to the surface and probes mechanical changes within the substrates. Unlike in previous combinations of these two single-molecule techniques [21] , [22] , [23] , [24] , we not only measure the intensity of individual fluorophores but also perform particle tracking of single fluorophore-labelled proteins [25] , [26] moving along a linear ssDNA track, stabilized with the aid of an optical trap. To illustrate the capacity of our instrument, we examined the ssDNA translocase and helicase activities of a superfamily 1 helicase, Escherichia coli UvrD. UvrD is a 3′–5′ DNA helicase involved in many DNA metabolic processes, such as mismatch repair [27] , nucleotide excision repair [28] and replication of certain plasmids [29] . The enzyme is also a 3′–5′ ssDNA translocase [30] , [31] , [32] , [33] , and the translocase activity is presumably required for its role as an anti-recombinase in which it displaces RecA protein filaments from ssDNA [34] , [35] to control potentially toxic recombination intermediates [6] . UvrD monomer translocation along ssDNA is highly processive, that is, the enzyme is estimated to translocate more than a thousand nucleotides before dissociating from DNA, although this estimate was based on ensemble kinetic studies performed using ssDNA up to ~100 nt long [30] , [31] . However, there have been conflicting reports about the oligomeric state of the active helicase in vitro , some claiming that a UvrD monomer can function as a processive helicase [36] , [37] , whereas others indicate that a monomer can translocate, yet a dimeric UvrD is required for processive helicase activity [30] , [35] , [38] , [39] , [40] . Although single-molecule force methods, such as magnetic tweezers, have revealed valuable information on the helicase activity of UvrD [41] , [42] , purely mechanical approaches cannot report on the ssDNA translocase activity in real time, because translocation does not change the overall length of DNA. Here the translocation of UvrD over thousands of nucleotides was visualized, providing the first demonstration of fluorescence imaging of single-protein movement on long ssDNA. In our experiments, a translocating monomeric UvrD stopped at a ssDNA/dsDNA junction, unable to unwind the duplex ahead. Moreover, with the unique capability of our instrument to probe both ssDNA translocase and helicase activities, we observe that at least two UvrD monomers are involved in DNA unwinding and can directly visualize the two unwinding initiation pathways proposed by a previous ensemble study [39] . Molecule-by-molecule analysis of translocation and unwinding rates provide strong constraints on the stepping mechanisms of UvrD during translocation and unwinding. Preparation of long ssDNA constructs In addition to overcoming the issue of ssDNA forming secondary structures, the preparation of pure, long ssDNA constructs with custom modifications (usually required for single-molecule force spectroscopy) poses additional technical challenges. Although asymmetric PCR [43] or terminal transferase reaction with deoxyribonucleotides can produce long ssDNA [44] with custom modifications at the 5′-end, the ssDNA product from these methods is a mixture of different lengths or sequences. To get higher-purity ssDNA constructs, dsDNA constructs can be produced with all the required modifications using standard PCR first, followed by subsequent removal of one strand from the constructs, via either overstretching [45] , chemical or thermal denaturation [46] , or exonuclease treatment [47] . To avoid base-pairing interactions between different ssDNA molecules, we immobilized the 5-kbp dsDNA (4,957 bp+1 nt) constructs on the surface before removing one strand. Once they are immobilized, spatial separation ensures that all the constructs are single DNA molecules even after they become single stranded. We used T7 exonuclease to digest one complementary strand away from the dsDNA constructs on the surface in situ . The dsDNA construct has a biotin label at the 5′-end of the UvrD tracking strand that is shielded by neutravidin binding, so only the 5′-end of the complementary strand is exposed to the 5′–3′ exonuclease. The reaction thus creates a partial duplex DNA with a dsDNA region near the surface and a 3′-ssDNA tail protruding away from the surface ( Fig. 1 and Supplementary Fig. S1 ). 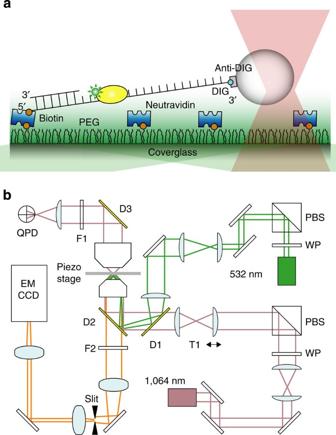Figure 1: Schematic and optical layout of the instrument. (a) Schematic of experimental setup. One end of a DNA construct is immobilized on the polyethylene glycol (PEG)-coated surface, and the other end is attached to a polystyrene bead confined in the optical trap (pink). Green excitation laser selectively illuminates molecules within a few hundred nanometres from the coverglass surface by TIR. (b) Optical layout of the instrument showing light pathways for 532-nm fluorescence excitation laser (green), 1,064-nm trapping laser (pink) and fluorescence emission (orange). The intensities of both the fluorescence excitation laser and the trapping laser are modulated by half wave plates (WP) and polarizing beam splitters (PBS). Two beams are combined at the dichroic mirror D1 and enter into the microscope. Trapping laser light scattered by a bead confined in the optical trap is imaged on to the quadrant photodiode detector (QPD) for monitoring the position of the trapped bead. The sample on the piezo stage is illuminated by objective-type TIRF, and the fluorescence emission is collected by an EMCCD (electron-multiplying charge-coupled device) camera. D1-3, dichroic mirrors; F1-2, filters; T1, a telescope. Figure 1: Schematic and optical layout of the instrument. ( a ) Schematic of experimental setup. One end of a DNA construct is immobilized on the polyethylene glycol (PEG)-coated surface, and the other end is attached to a polystyrene bead confined in the optical trap (pink). Green excitation laser selectively illuminates molecules within a few hundred nanometres from the coverglass surface by TIR. ( b ) Optical layout of the instrument showing light pathways for 532-nm fluorescence excitation laser (green), 1,064-nm trapping laser (pink) and fluorescence emission (orange). The intensities of both the fluorescence excitation laser and the trapping laser are modulated by half wave plates (WP) and polarizing beam splitters (PBS). Two beams are combined at the dichroic mirror D1 and enter into the microscope. Trapping laser light scattered by a bead confined in the optical trap is imaged on to the quadrant photodiode detector (QPD) for monitoring the position of the trapped bead. The sample on the piezo stage is illuminated by objective-type TIRF, and the fluorescence emission is collected by an EMCCD (electron-multiplying charge-coupled device) camera. D1-3, dichroic mirrors; F1-2, filters; T1, a telescope. Full size image For each DNA molecule, the lengths of both the 3′-ssDNA tail and duplex segment were estimated by fitting the force–extension curve of the molecule to the theoretical polymer models of ssDNA and dsDNA. We used the extensible worm-like chain model and extensible freely jointed chain model for dsDNA and ssDNA sections, respectively [45] , [48] . After 30 min of exonuclease treatment, 70% of the molecules had a ssDNA region longer than 3,500 nucleotides ( Supplementary Fig. S2 ). Visualization of ssDNA translocase activity of E. coli UvrD We measured ATP-driven translocation of E. coli UvrD along ssDNA. A schematic of the experimental set-up is shown in Fig. 1a . The long 3′-ssDNA tail of the DNA is the tracking strand on which the enzyme translocates in a 3′–5′ direction [30] , and the DNA is stretched by the optical trap. This scheme projects the enzyme motion along the strand onto a straight line. The angle between the stretched DNA construct and the surface is calculated as the arctangent of the height of a trapped bead (660 nm) to the lateral displacement of the trap centre from the 5′-end of DNA construct. Using this angle, we converted the distance projected on the surface to that of the stretched DNA construct, but this correction was less than 3% in most cases. For fluorescence imaging, UvrD was labelled with a single Cy3 molecule at residue 100 using a single cysteine mutant with 95% efficiency without compromising the enzyme’s function, as reported previously [49] . 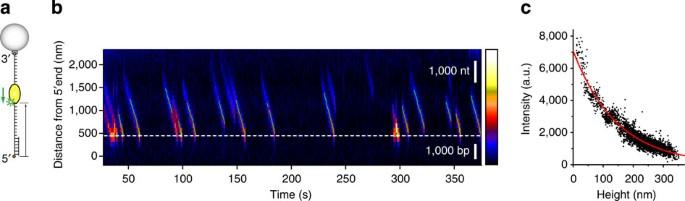Figure 2: Imaging UvrD translocation. (a) A partial duplex DNA construct with a long 3′-ssDNA tail. (b) A kymogram of multiple UvrD translocation events along a chosen DNA molecule stretched at 13.5 pN tension. Fluorescence intensity is colour-coded, and the colour scale is shown on the right (minimum intensity: balck (bottom); maximum intensity: white (top)). The translocation of UvrD follows a uniform motion and the speed of the translocation events are very similar, if not identical to each other. The estimated location of ssDNA/dsDNA junction is shown as the white dashed line, and the UvrD motion is observed exclusively in the ssDNA segment (above the white dashed line). Fitting the force–extension curve of this DNA molecule to the model (Supplementary Fig. S2) revealed that the length of dsDNA segment is ~1,370 bp, which is translated to 454 nm (where the dashed line is drawn) at 13.5 pN according to extensible worm-like chain model. Scale bars representing the length of 1,000 nt (ssDNA) and 1,000 bp (dsDNA) at 13.5 pN are shown in white. (c) Determination of the penetration depth of TIRF illumination. Fluorescence intensity is plotted against the height from the surface for selected translocation events at the same intensity of fluorescence excitation light (black). An exponential decay curve (red) is fit to the data to determine the penetration depth, 150 nm. Figure 2 presents a kymogram, which visualizes the time course of the fluorescence image at a glance. The kymogram shows the translocation activity along the 3′-ssDNA tail. UvrD monomers bind to a DNA molecule sequentially and translocate from the top (3′-end) to the bottom (5′-end), as expected for a 3′–5′ ssDNA translocase ( Supplementary Movie 1 ). Fluorescence emission intensity increases as UvrD approaches the 5′-end on the surface due to the increase in the excitation intensity in the TIR configuration. Fluorescence emission intensity decreases exponentially with the estimated height from the surface ( Fig. 2c ). By fitting the curve to an exponential decay, we estimated the penetration depth of the evanescent field excitation to be 150±30 nm. Figure 2: Imaging UvrD translocation. ( a ) A partial duplex DNA construct with a long 3′-ssDNA tail. ( b ) A kymogram of multiple UvrD translocation events along a chosen DNA molecule stretched at 13.5 pN tension. Fluorescence intensity is colour-coded, and the colour scale is shown on the right (minimum intensity: balck (bottom); maximum intensity: white (top)). The translocation of UvrD follows a uniform motion and the speed of the translocation events are very similar, if not identical to each other. The estimated location of ssDNA/dsDNA junction is shown as the white dashed line, and the UvrD motion is observed exclusively in the ssDNA segment (above the white dashed line). Fitting the force–extension curve of this DNA molecule to the model ( Supplementary Fig. S2 ) revealed that the length of dsDNA segment is ~1,370 bp, which is translated to 454 nm (where the dashed line is drawn) at 13.5 pN according to extensible worm-like chain model. Scale bars representing the length of 1,000 nt (ssDNA) and 1,000 bp (dsDNA) at 13.5 pN are shown in white. ( c ) Determination of the penetration depth of TIRF illumination. Fluorescence intensity is plotted against the height from the surface for selected translocation events at the same intensity of fluorescence excitation light (black). An exponential decay curve (red) is fit to the data to determine the penetration depth, 150 nm. Full size image Each translocating UvrD displayed a uniform velocity and the trajectories of different molecules in the kymogram are parallel, suggesting only a small variance in their speed of motion. The uniform brightness of moving fluorescent spots and a single-step photobleaching indicated that the translocating species is a UvrD monomer. We fitted fluorescence images to two-dimensional (2D) Gaussian functions ( Supplementary Fig. S3 ) and obtained the position and intensity trajectories of UvrD molecules ( Supplementary Fig. S4 ). For each translocation event, the position trajectory was fitted to a straight line to acquire the average translocation rate, and events that show more than one photobleaching step were discarded to limit the analysis to monomers of UvrD. At 1 mM ATP and 13.5 pN of force applied to the DNA, the enzymes translocated with a mean rate of 193 nt s −1 and s.d. of 22 nt s −1 ( Fig. 3a ). We also determined the distance translocated by the enzyme before abrupt disappearance of the fluorescence signal due either to photobleaching or enzyme dissociation from the DNA. By analysing the number of UvrD molecules still bound to DNA after translocating a given distance, we determined the apparent ssDNA translocation processivity to be 1,260±60 nt ( Fig. 3b ). However, the translocation distance may be underestimated due to the finite size of the illumination volume as well as fluorophore photobleaching. Dependence of the UvrD translocation rate on the tension applied to the DNA was minimal between 8 pN and 20 pN ( Fig. 3c ). Although a force-independent translocation rate was previously inferred via indirect methods for UvrD and other helicases [41] , [50] , [51] , our data represent the first direct demonstration of force independence of a helicase translocation on ssDNA. 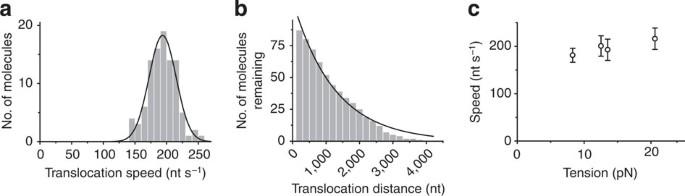Figure 3: Statistics of UvrD translocation. (a) Distribution of UvrD translocation speed fit to a Gaussian (black curve). The mean and s.d. of the distribution are 193 nt s−1and 22 nt s−1, respectively. (b) The number of molecules still remaining on DNA after translocating a given distance. The black curve is the fit to an exponential decay with a translocation processivity (the inverse of decay constant) of 1,260±60 nt. (c) The translocation speed was measured as a function of applied tension to DNA at a constant ATP concentration of 1 mM. The error bars correspond to s.d. The extension of one nucleotide under the applied tension was estimated using the extensible freely jointed chain model, and this length was used to convert the speed to nt s−1and distance to nt fora–c. Figure 3: Statistics of UvrD translocation. ( a ) Distribution of UvrD translocation speed fit to a Gaussian (black curve). The mean and s.d. of the distribution are 193 nt s −1 and 22 nt s −1 , respectively. ( b ) The number of molecules still remaining on DNA after translocating a given distance. The black curve is the fit to an exponential decay with a translocation processivity (the inverse of decay constant) of 1,260±60 nt. ( c ) The translocation speed was measured as a function of applied tension to DNA at a constant ATP concentration of 1 mM. The error bars correspond to s.d. The extension of one nucleotide under the applied tension was estimated using the extensible freely jointed chain model, and this length was used to convert the speed to nt s −1 and distance to nt for a – c . Full size image UvrD monomers stall at a ss/ds DNA junction Whether DNA unwinding can be carried out by a UvrD monomer has been the subject of some discussion. Transient kinetic ensemble studies have concluded that a dimeric UvrD species is needed for unwinding in vitro [30] , [35] , [38] , [39] , [42] , [52] , whereas others have concluded that a UvrD monomer is the unwinding species [36] , [37] . With our method, we can directly address this question by simply observing the enzyme as it encounters an ssDNA/dsDNA junction during ssDNA translocation. Although the majority of translocating UvrD displayed uniform motion along a straight line, some enzymes stopped translocation and stayed at a certain position (hereafter termed a ‘stall’) ( Fig. 4a ). When more than one stall event was observed on the same DNA, they occurred at the same location, and no other molecules translocated past that position. We suggest that the stall is caused by a structural blockade on the DNA, specifically the ssDNA/dsDNA junction. As the DNA construct consists of a dsDNA segment on the surface side and a long ssDNA 3′-tail on the other, UvrD molecules will encounter an ssDNA/dsDNA junction while moving along the tracking strand. If a UvrD monomer cannot unwind DNA, its forward progress will be prevented by the duplex junction and a stall would result, as we observed. To test this hypothesis, we plotted the distance between the stall position and the 5′-end of the tracking strand, determined via fluorescence imaging, against the length of the dsDNA segment for each DNA determined from a force–extension curve ( Fig. 4c ). We found a strong linear dependence with a slope of 1, implying that the stall location coincides with the ssDNA/dsDNA junction, supporting our interpretation that UvrD monomer translocation is blocked by the DNA double helix. To further test our interpretation, we designed another experiment such that we can determine the location of the ssDNA/dsDNA junction directly. An additional ssDNA/dsDNA junction was created by annealing a fluorescently labelled complementary oligodeoxynucleotide to the tracking strand, thus the position of the ssDNA/dsDNA junction can be determined by the fluorescence of the oligodeoxynucleotide ( Fig. 4d ). In Fig. 4e , a translocating UvrD monomer encounters the duplex region (indicated by the stationary Cy3 fluorescence) and stalls there until it photobleaches or dissociates. It is evident that the stalling position coincides with the stationary Cy3 fluorophore position. The distribution of the difference between stalling position and Cy3 position, presented in Fig. 4g , displays a sharp distribution around zero with an s.d. of 16 nm, indicating that stalling happens at the ssDNA/dsDNA junction. 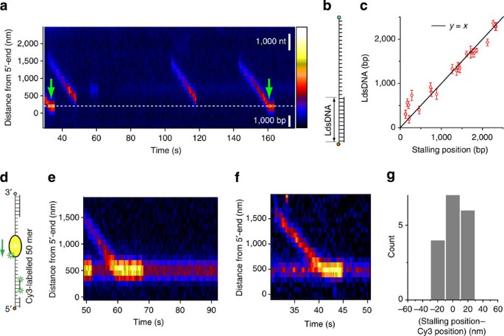Figure 4: UvrD translocation is blocked by dsDNA. (a) A kymogram showing stalling of UvrD. There is a certain location on a DNA where UvrD stops its translocation and stalls (green arrows). The stalling position is close to the white dashed line, which indicates the position of ssDNA/dsDNA junction (the length of duplex segment estimated from fitting the force–extension curve to the model). Scale bars correspond to the length of 1,000 nt (ssDNA) and 1,000 bp (dsDNA), respectively. (b) A partial duplex DNA construct used in the experiment is shown here. The length of duplex segment is estimated by fitting the force–extension curve to a polymer model. (c) The correlation between the length of duplex segment (the position of the junction) and the distance of the stalling position from the 5′-end of the tracking strand in the DNA constructs. The error bar represents the standard error. The scatter plot follows the identity relation (y=x,R2=0.95), which suggests that the stalling occurs at the ssDNA/dsDNA junction. (d) Another experiment designed to measure the location of ssDNA/dsDNA junction more directly. An additional ssDNA/dsDNA junction is created by annealing a fluorophore-labelled oligonucleotide to the tracking strand. We doubly labelled the oligonucleotide by way of precaution against fluorophore photobleaching. (e) A kymogram of a translocating UvrD monomer, eventually blocked by the presence of duplex region created by a complementary oligonucleotide annealed to the tracking strand. At ~52 s, one of the two fluorophores on the complementary oligonucleotide photobleaches, but the remaining Cy3 fluorophore marks the location of duplex region until the end of the kymogram. (f) Another kymogram showing UvrD stalling events. Here as well, translocation stops at the position of Cy3 fluorescence. (g) The distribution of the difference between stalling position and Cy3 position (the position of ssDNA/dsDNA junction) for 17 stalling events. Figure 4: UvrD translocation is blocked by dsDNA. ( a ) A kymogram showing stalling of UvrD. There is a certain location on a DNA where UvrD stops its translocation and stalls (green arrows). The stalling position is close to the white dashed line, which indicates the position of ssDNA/dsDNA junction (the length of duplex segment estimated from fitting the force–extension curve to the model). Scale bars correspond to the length of 1,000 nt (ssDNA) and 1,000 bp (dsDNA), respectively. ( b ) A partial duplex DNA construct used in the experiment is shown here. The length of duplex segment is estimated by fitting the force–extension curve to a polymer model. ( c ) The correlation between the length of duplex segment (the position of the junction) and the distance of the stalling position from the 5′-end of the tracking strand in the DNA constructs. The error bar represents the standard error. The scatter plot follows the identity relation ( y = x , R 2 =0.95), which suggests that the stalling occurs at the ssDNA/dsDNA junction. ( d ) Another experiment designed to measure the location of ssDNA/dsDNA junction more directly. An additional ssDNA/dsDNA junction is created by annealing a fluorophore-labelled oligonucleotide to the tracking strand. We doubly labelled the oligonucleotide by way of precaution against fluorophore photobleaching. ( e ) A kymogram of a translocating UvrD monomer, eventually blocked by the presence of duplex region created by a complementary oligonucleotide annealed to the tracking strand. At ~52 s, one of the two fluorophores on the complementary oligonucleotide photobleaches, but the remaining Cy3 fluorophore marks the location of duplex region until the end of the kymogram. ( f ) Another kymogram showing UvrD stalling events. Here as well, translocation stops at the position of Cy3 fluorescence. ( g ) The distribution of the difference between stalling position and Cy3 position (the position of ssDNA/dsDNA junction) for 17 stalling events. Full size image Moreover, a stalled UvrD at the junction did not unwind the DNA substrates to any detectable degree, as we did not observe any change in the end-to-end distance of the DNA in the force-based signal from the optical tweezers (our detection limit of DNA unwinding through force is about 25 bp, Supplementary Fig. S5b ). When a dsDNA molecule under tensions higher than ~6 pN is unwound, the end-to-end distance of the DNA increases because the extension per unit nucleotide is longer for ssDNA than for dsDNA [53] . As the optical trap position is fixed in our experiment, we expect to see a decrease in tension for the DNA molecules undergoing unwinding, but such tension changes were not observed. We cannot rule out the occurrence of unwinding events shorter than 25 bp that cannot be detected by this instrument. Ensemble kinetic experiments also do not detect UvrD monomer-catalysed unwinding of dsDNA as short as 18 bp [30] , [38] . Visualization of unwinding initiation pathways We could still observe, albeit rarely, unwinding of the dsDNA segments even at the low UvrD concentrations we had to use to resolve single UvrD molecules (100–200 pM). For each unwinding event, we could monitor the position of UvrD molecules (via fluorophore tracking) and the number of UvrD monomers in the same fluorescent spot (via fluorescence intensity and photobleaching step counting) as they bind to the ssDNA segment, translocate down to the ssDNA/dsDNA junction, unwind the dsDNA segment and dissociate from the DNA end. In addition, by using optical tweezers we monitored the unwinding activity. The versatility of the method allowed us to observe directly the whole process of unwinding initiation and to distinguish two different pathways proposed previously based on ensemble kinetic studies [39] . 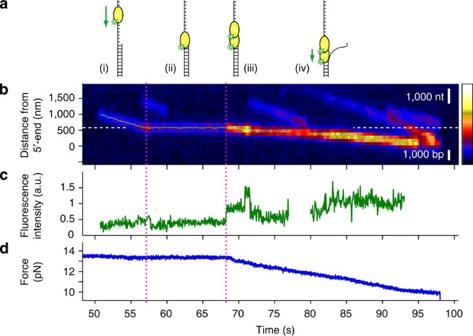Figure 5: The duplex DNA segment blocking translocation of UvrD is unwound as another UvrD binds to the junction. (a) Schematic drawings of this unwinding event: (i) one UvrD translocates until it encounters an ssDNA/dsDNA junction; (ii) it stops at the junction; (iii) the second UvrD binds to the junction; and (iv) the helicase unwinds the duplex DNA. (b) A kymogram of this event. White dashed line indicates the projected location of the junction. UvrD stalls at the junction for 15 s. At 68 s (magenta dotted line), there is a sudden increase in fluorescence intensity, followed by resumed UvrD motion, at a slower rate. The position trajectories from the 2D Gaussian fit are overlaid on top (light green). Scale bars for the length of 1,000 nt (ssDNA) and 1,000 bp (dsDNA) at 13.5 pN are shown in white. (c) The fluorescence intensity trajectory. At 68 s (magenta dotted line), there is a sudden increase in fluorescence, which designates the binding event of another UvrD. There is a third binding event (71 s) followed by quick dissociation (or photobleaching, 72 s), but this event does not seem to have a role in unwinding. (d) The force (tension in the DNA substrate) trajectory. The force is stable at 13.5 pN initially, which means no length change in the DNA substrate. At the second magenta dotted line, the force starts to decrease, which is the signature of dsDNA unwinding. Figure 5 ( Supplementary Movie 2 ) shows an example set of data in which one UvrD monomer translocates in the 3′–5′ direction along the ssDNA section and stalls at the ssDNA/dsDNA junction. After 15 s, another UvrD monomer from the solution binds as is apparent from the sudden increase in fluorescence intensity by a factor of two. Simultaneously, within our measurement uncertainty of 0.3 s, unwinding is initiated as reported by a gradual decrease in tension and by the movement of the UvrD molecules towards the surface at a significantly reduced speed compared with the translocation speed on the ssDNA tail (67 bp s −1 , threefold slower than the ssDNA translocation). This is consistent with ensemble-transient kinetic measurements in which DNA unwinding by UvrD is known to be slower by threefold compared with ssDNA translocation [30] . Thus, a stalled UvrD monomer at the ssDNA/dsDNA junction is joined by a second UvrD monomer and unwinding is initiated. The second UvrD monomer can also bind to the ssDNA tail, translocate to the junction and join the stalled UvrD to initiate unwinding ( Supplementary Fig. S6 ). Recruitment of a second UvrD to a stalled UvrD, either directly from solution or via ssDNA translocation, represents the first of the two pathways of DNA unwinding initiation proposed previously [39] . Figure 5: The duplex DNA segment blocking translocation of UvrD is unwound as another UvrD binds to the junction. ( a ) Schematic drawings of this unwinding event: (i) one UvrD translocates until it encounters an ssDNA/dsDNA junction; (ii) it stops at the junction; (iii) the second UvrD binds to the junction; and (iv) the helicase unwinds the duplex DNA. ( b ) A kymogram of this event. White dashed line indicates the projected location of the junction. UvrD stalls at the junction for 15 s. At 68 s (magenta dotted line), there is a sudden increase in fluorescence intensity, followed by resumed UvrD motion, at a slower rate. The position trajectories from the 2D Gaussian fit are overlaid on top (light green). Scale bars for the length of 1,000 nt (ssDNA) and 1,000 bp (dsDNA) at 13.5 pN are shown in white. ( c ) The fluorescence intensity trajectory. At 68 s (magenta dotted line), there is a sudden increase in fluorescence, which designates the binding event of another UvrD. There is a third binding event (71 s) followed by quick dissociation (or photobleaching, 72 s), but this event does not seem to have a role in unwinding. ( d ) The force (tension in the DNA substrate) trajectory. The force is stable at 13.5 pN initially, which means no length change in the DNA substrate. At the second magenta dotted line, the force starts to decrease, which is the signature of dsDNA unwinding. Full size image When the concentration of UvrD is increased to 1 nM, we observe a second unwinding initiation pathway ( Fig. 6 ). Multiple UvrD molecules translocate on the substrate together as a single spot until arriving at the ssDNA/dsDNA junction. They consist of at least two UvrD monomers, because the fluorescence intensity decreases in two steps and the original intensity is about twofold higher than the intensity of a UvrD monomer ( Fig. 6 ). They do not stall at the junction, but instead proceed to unwind the duplex substrate, although at a much slower rate relative to translocation (14 bp s −1 for the event in Fig. 6 ). Dissociation of the enzyme from the unwound dsDNA leads to a sudden decrease in fluorescence intensity and a concurrent increase in tension in the force-time trajectory due to immediate rezipping of duplex DNA. Unlike the narrow distribution of the translocation rates, the unwinding rate displays a broad distribution with a mean of 70 bp s −1 and an s.d. of 31 bp s −1 , respectively (32 unwinding events, Supplementary Fig. S7 ). 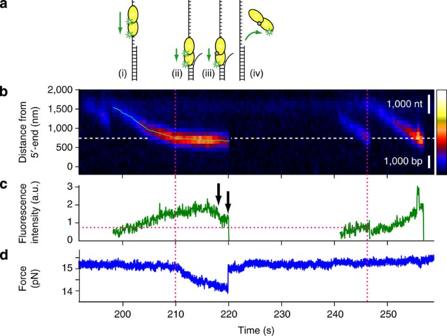Figure 6: Two UvrD molecules translocate together and unwind the duplex segment without stalling. (a) Schematic of this unwinding event: (i) two UvrD molecules translocate together toward the ssDNA/dsDNA junction; (ii) they proceed and unwind the junction without a pause; (iii) one fluorophore photobleaches, but the helicase keeps unwinding; and (iv) as they dissociate, the unwound duplex is immediately rezipped. (b) A kymogram of this unwinding event. White dashed line designates the estimated location of the ssDNA/dsDNA junction. Although it looks like a stalling, the position trajectory obtained from 2D Gaussian fitting (light green) reveals a slow forward motion, as expected for unwinding. For the fluorescence intensity comparison, other UvrD molecules were included. (c) The fluorescence intensity trace of the event proves that there are at least two fluorescent dyes, that is, two UvrD monomers involved in this unwinding event. First, there are two fluorescence decrease steps (black arrows). Second, the intensity of UvrD in this event is twofold higher than the intensity of another UvrD near the junction (magenta dotted lines). (d) The force trajectory. The force starts to decrease as UvrD reaches the junction (magenta dotted line). The dissociation of the enzyme from the substrate (the second black arrow) causes the duplex to rezip immediately. Figure 6: Two UvrD molecules translocate together and unwind the duplex segment without stalling. ( a ) Schematic of this unwinding event: (i) two UvrD molecules translocate together toward the ssDNA/dsDNA junction; (ii) they proceed and unwind the junction without a pause; (iii) one fluorophore photobleaches, but the helicase keeps unwinding; and (iv) as they dissociate, the unwound duplex is immediately rezipped. ( b ) A kymogram of this unwinding event. White dashed line designates the estimated location of the ssDNA/dsDNA junction. Although it looks like a stalling, the position trajectory obtained from 2D Gaussian fitting (light green) reveals a slow forward motion, as expected for unwinding. For the fluorescence intensity comparison, other UvrD molecules were included. ( c ) The fluorescence intensity trace of the event proves that there are at least two fluorescent dyes, that is, two UvrD monomers involved in this unwinding event. First, there are two fluorescence decrease steps (black arrows). Second, the intensity of UvrD in this event is twofold higher than the intensity of another UvrD near the junction (magenta dotted lines). ( d ) The force trajectory. The force starts to decrease as UvrD reaches the junction (magenta dotted line). The dissociation of the enzyme from the substrate (the second black arrow) causes the duplex to rezip immediately. Full size image We have demonstrated direct fluorescence imaging of protein dynamics on long ssDNA using E. coli UvrD helicase/translocase. We were able to probe the whole series of events for UvrD interaction with a DNA substrate, including binding, ssDNA translocation, DNA unwinding (helicase activity) and dissociation at a single-protein resolution. To measure the ssDNA translocation rate and processivity of UvrD monomers, we used very low concentrations of UvrD. At 100–200 pM concentrations, the majority of UvrD molecules observed are monomers, as the fraction of UvrD dimers in solution is well below 0.1% [54] . Direct measurement yielded a UvrD monomer ssDNA translocation rate of 193 (±2) nt s −1 , which coincides with the values determined from ensemble experiments on oliogodeoxythymidylates [30] , [31] , [32] under similar conditions (10 mM Tris–HCl (pH 8.3), 20 mM NaCl, 20% (v/v) glycerol, 1 mM ATP:Mg 2+ at 25 °C). These ensemble experiments estimated the processivity of ssDNA translocase activity of UvrD to be 769 nt in the presence of a heparin trap [31] and 2,400 (±600) nt in the absence of a competing trap [30] , which are much longer than the length of ssDNA molecules (10–124 nt) used, whereas in our experiments individual translocation events as long as thousands of nucleotides were directly observed ( Fig. 3b ). Although our measured value of the ssDNA translocation processivity, 1,260 (±60) nt, is likely to be an underestimation, it falls between the two previous measurements. The ssDNA translocase activity of a UvrD monomer is so processive that even 4,000 nt is not long enough to eliminate an effect of the finite size of ssDNA molecules on the processivity estimate. Ensemble-transient kinetics studies have yielded information on a multitude of kinetic properties of the ssDNA translocase activity and DNA unwinding activity of UvrD, including the kinetic step size [30] , [31] , [32] , [33] , [52] , [55] . However, the kinetic step size estimation can be complicated by the presence of static disorder (persistent heterogeneity) that can result in significant molecule-to-molecule differences in the translocation rates within the ensemble population [6] , [33] . For example, the kinetic ssDNA translocation step size of E. coli PcrA, a SF1 helicase and ssDNA translocase that shares extensive structural and sequence similarity with E. coli UvrD, was determined to be 1 nt in single-molecule experiments [6] , whereas ensemble assays estimated it to be 4–5 nt [56] . The overestimation in the latter experiments was attributed to persistent heterogeneity observed in the translocation rate of single PcrA molecules [6] . To assess the molecular heterogeneity of UvrD, we examined the distribution of the rates of multiple UvrD molecules that translocated on the same DNA, to exclude DNA-to-DNA variation ( Fig. 7 ). The distribution displayed a small dispersion, as the coefficient of variation was 10%, which was smaller than the 22% observed for the translocation rate of PcrA [6] . Therefore, the ~4 nt kinetic step size estimated for UvD monomer translocation and the resulting proposal of a non-uniform stepping mechanism [31] , [33] cannot be attributed to molecular heterogeneity. 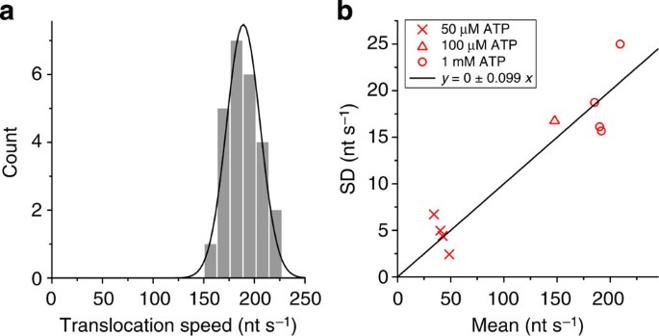Figure 7: Molecular heterogeneity in the translocation rate of a monomeric UvrD translocase. (a) The distribution of translocation rates of 28 UvrD molecules on the same DNA substrate (the substrate inFig. 2) shown with the Gaussian fit (black). The mean and s.d. are 189 nt s−1and 17 nt s−1, respectively. The spread in this distribution only consists of the measurement error and the molecular heterogeneity, because all events were recorded on the same DNA substrate. (b) For the DNA substrates that had more than eight UvrD translocation events, the mean and the s.d. of the translocation rate are plotted (red). The black line is the linear fit of the data, which yields the coefficient of variation (the ratio of the s.d. to the mean) of 0.10. Figure 7: Molecular heterogeneity in the translocation rate of a monomeric UvrD translocase. ( a ) The distribution of translocation rates of 28 UvrD molecules on the same DNA substrate (the substrate in Fig. 2 ) shown with the Gaussian fit (black). The mean and s.d. are 189 nt s −1 and 17 nt s −1 , respectively. The spread in this distribution only consists of the measurement error and the molecular heterogeneity, because all events were recorded on the same DNA substrate. ( b ) For the DNA substrates that had more than eight UvrD translocation events, the mean and the s.d. of the translocation rate are plotted (red). The black line is the linear fit of the data, which yields the coefficient of variation (the ratio of the s.d. to the mean) of 0.10. Full size image In contrast to the ssDNA translocation rates of the UvrD monomer, the distribution of unwinding rates for the dimeric UvrD helicase under 13.5 pN applied tension was broad with mean and s.d. of 70 bp s −1 and 31 bp s −1 , respectively. The rate agrees well with the ensemble DNA unwinding rate measurement of 68 (±9) bp s −1 (ref. 38 ), but differs significantly from the 248 (±74) bp s −1 rate reported from a magnetic tweezers experiment at 35 pN [41] . In fact, as discussed previously [30] the unwinding rate from the latter is closer to the ssDNA translocation rate measured here and previously [30] , suggesting that the ssDNA translocase activity alone might be enough to unwind dsDNA if high tension is applied on the tracking DNA strand. Another magnetic tweezers experiment [42] reported that UvrD unwinding rates decreased with an increase of force applied in the direction of strand separation and the unwinding rate at zero force was 60 (±7) bp s −1 . The rate at zero force is relevant to our case wherein tension is not applied in the unzipping direction, and is in agreement with our measurement within error. A previous ensemble kinetic study on DNA unwinding by UvrD estimated 4–5 bp of kinetic step size [55] . Because of the heterogeneity in unwinding rate between single DNA molecules, which can inflate the estimated kinetic step size [6] , it is possible that the true kinetic step size is lower than 4–5 bp. A single DNA unwinding analysis of UvrD also estimated the kinetic step size to be about 4–5 bp, but their analysis based on variance analysis as used in ensemble kinetic studies can also be influenced by persistent molecular heterogeneity [41] . Direct measurements of unwinding step size using high-resolution single-molecule assays [57] , [58] , [59] are needed to address the issue of the step size during DNA unwinding. The large contrast between the homogenous ssDNA translocation rate and the inhomogeneous DNA unwinding rate is unexpected. The homogeneous ssDNA translocation rate of single UvrD molecules show that there is little heterogeneity in the activities of single proteins. Nevertheless, when more than one UvrD protein collaborates to unwind dsDNA, there is a large heterogeneity in the unwinding rate, suggesting that DNA unwinding is not always done by a single species in a single active conformation. We also observed that UvrD monomer translocation stops upon encountering a ssDNA/dsDNA junction and does not proceed further. The fact that translocating UvrD monomers do not make a transition to unwinding duplex DNA but stop at the junction indicate that the translocase and helicase activities of UvrD are separable and that both activities may be used selectively for different processes in vivo [35] . These results also highlight the fact that UvrD self-assembly regulates its helicase activity in vitro [35] , as UvrD monomers stalled at the junction never initiate unwinding on their own, even after long pauses. Ensemble-transient kinetic studies [39] have suggested that there are two pathways leading to the formation of the active UvrD helicase–DNA complex. Here we directly visualized these two pathways for initiation of DNA unwinding at the single-molecule level. In the first pathway, a translocating UvrD monomer, blocked by the ssDNA/dsDNA junction, stalls and pauses until another UvrD molecule is recruited to the junction to activate helicase activity and unwind duplex DNA. In the second, two or more UvrD monomers translocate together along ssDNA at the same translocation speed of monomers until they encounter the ssDNA/dsDNA junction and then proceed to unwind dsDNA. The observation of simultaneous translocation of two monomers of UvrD as a single unit ( Supplementary Fig. S8 ) provides evidence for the existence of a translocating dimeric species of UvrD, rather than two independent monomers. Our method can be straightforwardly extended to multi-colour excitation and detection, to RNA substrates and to single-molecule FRET analysis. With such improvements, this method may be used to study the coordination of many proteins interacting on the same ss and ds DNA or RNA. Instrument design details Figure 1b shows the optical layout of the experimental set-up. The instrument is built based on an inverted microscope (Olympus IX71), with slight modification to mount a condenser and a dichroic mirror (D3) more stably. A sample is held horizontally on top of a XYZ piezo-nanostage (Mad City Labs) mounted on a manual stage (Semprex) with two micrometres in the x and y axis, which is fixed on top of the microscope. An oil-immersion objective lens ( × 100/1.40, Olympus) is used for objective-type TIRF microscopy and optical trapping. Only the vicinity of the coverglass—water interface of the sample chamber is excited by 532-nm diode-pumped solid state laser (Spectra Physics) for fluorescence excitation, and fluorescence emission is imaged onto an EMCCD (electron-multiplying charge-coupled device) camera (Andor iXon) and is recorded at the frame rate of 20 Hz. At the centre of the fluorescence imaging area, an optical trap is formed a using collimated 1,064-nm Nd-YAG laser (Spectra Physics). Antidigoxigenin-coated polystyrene beads (Spherotech; 880 nm in diameter) are used for optical trapping. The focus of the trapping laser is adjusted to make the bottom of a trapped bead very close to the surface of the sample chamber (<250 nm from the coverslip) to ensure that the majority of DNA stretched by the trap is placed within the penetration depth of fluorescence excitation. Scattered laser light from a trapped bead is collected by condenser lens and imaged onto a quadrant photodiode detector (Pacific Sensors). More details on the instrument design, calibration and operation are available in Supplementary Methods . Preparation of DNA constructs The dsDNA (4,957 bp) constructs were synthesized by using PCR, using a biontinylated primer and a regular primer ( Supplementary Fig. S1a ). The PCR product encompassed the sequence (19,360, 24,316) from bacteriophage λ DNA (New England Biolabs). Purified PCR products were incubated with terminal transferase (New England Biolabs) and digoxigenin-11-dideoxyUTP (Roche Applied Science) to label 3′-ends of the PCR product with a single digoxigenin-modified digoxigenin-11-dideoxyUTP ( Supplementary Fig. S1b ) to attach this end to antidigoxigenin-coated beads. After the 5-kbp dsDNA (4,957 bp+1 nt) constructs are immobilized on the surface, T7 exonuclease (New England Biolabs) is injected into the chamber ( Supplementary Fig. S1c ). Because of the biotin–neutravidin coupling on the 5′-end of one strand, the only available initiation site is the 5′-end of the complementary strand, thus, only the latter strand is selectively digested ( Supplementary Fig. S1d ). After the reaction, a partial duplex with long 3′-ssDNA tail ( Supplementary Fig. S1e ) or a fully ss ( Supplementary Fig. S1f ) DNA construct is generated. The length of the duplex region can be controlled by the incubation time of the exonuclease reaction. Finally, the antidigoxigenin-coated beads are added to the chamber to attach the beads to the 3′-end of the undigested strand of DNA constructs. (In principle, the beads can attach to digoxigenin on the 3′-end of the digested strand, too. However, with the digoxigenin on the strand being so close to the surface, it seems that it is very unlikely: we did not have the problem.) A different DNA construct was used in the UvrD stalling experiments presented in Fig. 4d–g . Two dsDNA PCR products (6,841 bp and 1,170 bp) are synthesized from the sequence (33,498, 40,338) and (12,176, 13,345) of bacteriophage λ DNA. The longer product has a biotin at one end, whereas the shorter product is phosphorylated on one end and digoxigenin-labelled on the other. The two products are ligated using T4 DNA ligase (New England Biolabs). After the construct is immobilized on the surface, the longer product part is digested using T7 exonuclease to provide long ssDNA track for UvrD translocation, whereas the shorter product part serves as a dsDNA handle that is attached to a trapped bead. A complementary oligonucleotide (5′-/Cy3/GCC GGA ACA GTA CGA CGA AAA GCC GCA GGT ACA GCA GGT AGC GCA GAT CA/Cy3/-3′) is annealed to the tracking ssDNA. Polymer modelling To estimate the length of dsDNA stem and the ssDNA tail in DNA substrates, we fit the force–extension relation of the substrate to standard theoretical model of DNA. The extension of the substrate is treated as the sum of the extension from its dsDNA and ssDNA segment [53] . For the dsDNA segment, we used the extensible worm-like chain model with a persistence length of 53 nm, a stretch modulus of 1,200 pN and a contour length of one dsDNA base pair of 0.34 nm [48] . For the ssDNA segment, we used the extensible freely jointed chain model with a persistence length of 0.75 nm, a stretch modulus of 800 pN and a contour length of one ssDNA nucleotide of 0.59 nm [45] . Experimental solution conditions All UvrD experiments were performed in 20 mM Tris–HCl (pH 8.3), 10 mM NaCl and 5 mM MgCl 2 at 24 °C. The concentration of UvrD monomers was varied between 100 pM–1 nM, and the ATP concentration was fixed at 1 mM. To enhance the stability and longevity of Cy3, we use 3 mM Trolox (Sigma-Aldrich), 0.8% dextrose with glucose oxidase (Sigma-Aldrich) and catalase (Calbiochem) [60] . How to cite this article: Lee, K. S. et al. Direct imaging of single UvrD helicase dynamics on long single-stranded DNA. Nat. Commun . 4:1878 doi: 10.1038/ncomms2882 (2013).